Intercalated architecture of MA2Z4family layered van der Waals materials with emerging topological, magnetic and superconducting properties The search for new two-dimensional monolayers with diverse electronic properties has attracted growing interest in recent years. Here, we present an approach to construct MA 2 Z 4 monolayers with a septuple-atomic-layer structure, that is, intercalating a MoS 2 -type monolayer MZ 2 into an InSe-type monolayer A 2 Z 2 . We illustrate this unique strategy by means of first-principles calculations, which not only reproduce the structures of MoSi 2 N 4 and MnBi 2 Te 4 that were already experimentally synthesized, but also predict 72 compounds that are thermodynamically and dynamically stable. Such an intercalated architecture significantly reconstructs the band structures of the constituents MZ 2 and A 2 Z 2 , leading to diverse electronic properties for MA 2 Z 4 , which can be classified according to the total number of valence electrons. The systems with 32 and 34 valence electrons are mostly semiconductors. Whereas, those with 33 valence electrons can be nonmagnetic metals or ferromagnetic semiconductors. In particular, we find that, among the predicted compounds, (Ca,Sr)Ga 2 Te 4 are topologically nontrivial by both the standard density functional theory and hybrid functional calculations. While VSi 2 P 4 is a ferromagnetic semiconductor and TaSi 2 N 4 is a type-I Ising superconductor. Moreover, WSi 2 P 4 is a direct gap semiconductor with peculiar spin-valley properties, which are robust against interlayer interactions. Our study thus provides an effective way of designing septuple-atomic-layer MA 2 Z 4 with unusual electronic properties to draw immediate experimental interest. Monolayer two-dimensional (2D) materials have attracted tremendous interest for their unique electronic properties distinct from corresponding bulk phases, which show promising potential in a variety of fields such as energy storage and conversion [1] , [2] , nanoelectronics [3] , [4] , spintronics [5] , [6] , and superconductivity [7] , [8] , [9] , [10] , [11] , [12] , [13] , [14] , [15] , [16] . The electronic properties are strongly related to their geometric structures, which can be classified by the number of atomic layers ( n ). Up to now, most of the discovered monolayer 2D materials have a thickness with n ≤ 7. Graphene and hexagonal boron nitride ( h -BN) monolayer are famous six-membered ring (SMR) materials [17] of n = 1, which have been a central topic for over a decade [18] , [19] , [20] , [21] , [22] , [23] , [24] , [25] , [26] . In the silicon counterpart of graphene, the hexagonal honeycomb tends to be buckled into a double-atomic layer structure, that is, n = 2 (see Fig. 1 a) [27] . As for n = 3, monolayer transition-metal dichalcogenides (TMDs) are the most studied SMR materials [28] , [29] . In particular, 1 \({T}^{\prime}\) -WTe 2 monolayer is predicted to be a quantum spin Hall insulator [30] , [31] . Another popular system of n = 3 is the 2D ferromagnetic semiconductor CrI 3 , of which the magnetism can be manipulated by external electric fields and electrostatic dopings [32] , [33] , [34] . Among the family of n = 4, the monolayer group III chalcogenides have accepted growing interest. For instance, the semiconducting monolayer InSe exhibits extraordinary photocatalytic properties [35] . A strong electron–phonon coupling (EPC) can be obtained by an appropriate hole doping for this system, leading to interesting optical and transport properties [36] , [37] . The topological insulator Bi 2 Se 3 and 2D ferromagnetic semiconductor CrGeTe 3 are two representative systems of n = 5 [38] , [39] , [40] . Recently, CaMg was found to have a sextuple layer ( n = 6) structure [41] . Fig. 1: Geometric structures of known monolayer 2D materials and new MA 2 Z 4 monolayer materials. a Top and side views of representative monolayers for n ≤ 7, all belonging to the SMR materials [17] . b Schematic illustration of the intercalation method that uses the structures of a MoS 2 -like monolayer (2 H - and 1 T phases) and those of an InSe-like monolayer ( α and β phases) to construct the structures of a MA 2 Z 4 monolayer. Full size image The exploration of monolayer 2D materials has been extended to septuple layer systems in recent years. For instance, a ferromagnetic semiconducting monolayer of MnBi 2 Te 4 (Fig. 1 a) can be obtained from its antiferromagnetic bulk phase, which has nontrivial topological properties [42] , [43] , [44] , [45] . More recently, we experimentally synthesized a new compound of septuple layer SMR material, that is, MoSi 2 N 4 (see Fig. 1 a), which has a bandgap of ~1.94 eV with excellent ambient stability [46] . The geometric structures of these materials can be related to other layered systems. For instance, the structure of the MnBi 2 Te 4 monolayer can be viewed as an intercalated structure that is formed by inserting a single layer of the (111) plane MnTe ( n = 2) into a Bi 2 Te 3 monolayer ( n = 5) [47] . Likewise, the MoSi 2 N 4 monolayer can be built by intercalating a 2 H -MoS 2 -type MoN 2 layer ( n = 3) into an α -InSe-type Si 2 N 2 ( n = 4). As illustrated in Fig. 1 a, we have summarized these known monolayer 2D SMR materials consisting of n = 1, 2, 3, 4, 5, 6, and 7 atomic layer thicknesses. With varying n number, compositions, and constituents, they will become richer in both structures and properties. However, the difficulties lie in how we effectively seek for more monolayer materials with unusual electronic properties. Here, we have proposed a general intercalated architecture approach to systemically construct the structures of MA 2 Z 4 monolayers for the n = 7 family. We illustrate this scheme using density functional theory (DFT) calculations. In addition to reproducing the experimentally synthesized α 1 -MoSi 2 N 4 , α 1 -WSi 2 N 4 , and β 5 -MnBi 2 Te 4 monolayer materials, we also predict 70, thermodynamically and dynamically, stable MA 2 Z 4 monolayer materials, which exhibit diverse electronic properties including nontrivial topological properties, 2D ferromagnetism, Ising superconductivity, and robust electron valleys. Intercalated architecture approach We construct the structures of hexagonal MA 2 Z 4 monolayers by intercalating a MoS 2 -type MZ 2 layer into an InSe-type A 2 Z 2 monolayer, that is, the MZ 2 layer is sandwiched between two AZ layers. We consider two types of phases for each constituent, that is, the 2 H and 1 T phases for the hexagonal MZ 2 and the α and β phases for the A 2 Z 2 monolayer. Each type of the combinations of MZ 2 and A 2 Z 2 involves one pair of the phases. We note that on each side of the MZ 2 layer, there are three high-symmetry sites for both A and Z atoms in the AZ layers. Therefore, there are 36 configurations for each combination of MZ 2 and A 2 Z 2 . As a result, there are 144 possible configurations for each compound. We reduce the number of structures to 39 by removing the duplicated structures based on a symmetry analysis. In addition, we found that, among them, nine configurations are energetically unfavorable. 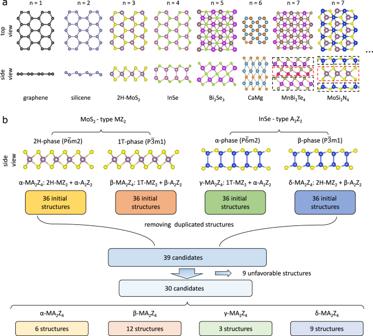Fig. 1: Geometric structures of known monolayer 2D materials and new MA2Z4monolayer materials. aTop and side views of representative monolayers forn≤ 7, all belonging to the SMR materials17.bSchematic illustration of the intercalation method that uses the structures of a MoS2-like monolayer (2H- and 1Tphases) and those of an InSe-like monolayer (αandβphases) to construct the structures of a MA2Z4monolayer. Therefore, we have considered 30 structures (Supplementary Table 1 ) for our first-principles calculations for each compound, which can be classified into four types, that is, α , β , γ , and δ respectively (see Fig. 1 b). As a benchmark, we first apply the scheme to MnBi 2 Te 4 , MoSi 2 N 4 , and WSi 2 N 4 . Our calculations found that the β 5 phase has the lowest energy for MnBi 2 Te 4 , which is exactly the structure of a single MnBi 2 Te 4 layer in the bulk phase [42] , [43] , [44] , [48] . For MoSi 2 N 4 and WSi 2 N 4 , our results reveal that the α 1 phase is the most stable structure, in agreement with our previous experiments [46] . Moreover, we have applied a structure prediction method RG 2 to search for possible structures for MoSi 2 N 4 and WSi 2 N 4 [49] . As a result, the predicted low-energy structures are within the 30 candidates. These results demonstrate the validity of our strategy in predicting monolayers with a septuple-atomic-layer structure. Energetics and stability of MA 2 Z 4 monolayers We now investigate the energetics and stability of MA 2 Z 4 monolayers. We have performed calculations for MA 2 Z 4 (M = elements of transition-metal groups IVB, VB, and VIB; A = Si, and Ge; and Z = N, P, and As). There are 54 compounds for this type of material, which have a number of valence electrons ranging from 32 to 34. Moreover, we have also carried out calculations for MA 2 Z 4 monolayers (M = alkali-earth group elements Mg, Ca, and Sr and group IIB elements Zn, Cd, and Hg; A = Al and Ga; and Z = S, Se, and Te). There are 36 compounds in this family, which have a number of 32 valence electrons. In Fig. 2 a, b, we show the enthalpies of formation of the five lowest-energy structures for each compound, for which the total energies of the α 1 and β 1 phases are used as the reference, respectively. More information about the enthalpies of formation and structural properties can be found in Supplementary Tables 2 – 7 . We found that the β 2 phase has the lowest energy for all the 32-electron systems, with M being the transition-metal group elements. The trends for the systems with 33 and 34 valence electrons are different. For MSi 2 N 4 (M = V, Nb, Ta, Cr, Mo, W), MGe 2 N 4 (M = Nb, Ta, Mo, W), and MSi 2 P 4 (M = Nb, Ta), the α 1 phase is the lowest-energy structure, whereas for MSi 2 P 4 (M = Cr, Mo, W), MGe 2 P 4 (M = V, Nb, Ta, Cr, Mo, W), and M(Si/Ge) 2 As 4 (M = V, Nb, Ta, Mo, W), the α 2 phase is found to be energetically lower than the others. We further investigate their stability by performing phonon calculations, for which the results are summarized in Supplementary Fig. 1 . Our calculations suggest that among the studied systems, with M being the transition-metal group elements, there are 48 compounds dynamically stable. The other six compounds, that is, β 2 -TiSi 2 N 4 , β 2 -TiGe 2 N 4 , β 2 -VGe 2 N 4 , β 2 -CrGe 2 N 4 , β 1 -CrSi 2 As 4 , and CrGe 2 As 4 , may be dynamically unstable since they exhibit imaginary phonon branches. Fig. 2: DFT-derived enthalpies of formation of MA 2 Z 4 monolayers. Here, we only show the data for the five lowest-energy configurations. a and b are for M being the first transition-metal group elements and alkali-earth elements, respectively. In a , b , the enthalpies for each compound are relative to the total energies of the α 1 and β 1 structures, respectively. Note that VEC is the number of valence electrons for one chemical formula. For more details about enthalpies of formation refer to Supplementary Tables 2 – 7 . Full size image The monolayers based on the alkali-earth group and group IIB elements are in either the β 1 or β 2 phase. Twenty-four compounds are expected to be stable based on the phonon calculations (Supplementary Fig. 2 ). It should be mentioned that four of them, that is, β 1 -ZnAl 2 S 4 , β 1 -ZnGa 2 S 4 , β 1 -MgAl 2 S 4 , and β 1 -MgAl 2 Se 4 , can be found from the 2DMatPedia database, which was obtained by the high-throughput computational method [41] . This agreement again indicates the validity of our intercalation method in predicting structures of the MA 2 Z 4 monolayers. Moreover, we have performed ab initio molecular dynamics simulations for selected systems, that is, β 2 -SrGa 2 Te 4 , δ 4 -VSi 2 P 4 , α 1 -TaSi 2 N 4 , and α 2 -WSi 2 P 4 (Supplementary Fig. 3 ), whose electronic properties will be discussed below. Our results indicate that they are thermally stable. In all, we have predicted 72 new monolayer materials with a septuple-atomic-layer structure. Electronic properties The intercalation method leads us to find a series of septuple layer MA 2 Z 4 materials with diverse electronic properties, summarized in Supplementary Figs. 4 – 7 , which are distinctly different from those of the constituents MZ 2 and A 2 Z 2 . For instance, the 2 H -NbN 2 monolayer is a metallic ferromagnet, while α -Si 2 N 2 is a semiconductor. However, the intercalated system α 1 -NbSi 2 N 4 is surprisingly a ferromagnetic semiconductor (Supplementary Fig. 5 ). We found that the electronic properties of MA 2 Z 4 can be classified according to the total number of valence electrons of these systems. The MA 2 Z 4 nitrides with 32 valence electrons are semiconductors. However, their phosphides and arsenides with such a number of valence electrons are metallic, which is due to a much weaker band hybridization between the M and Z atoms in these systems than in the nitrides. Most of the MA 2 Z 4 systems with 34 valence electrons are semiconductors, except for CrGe 2 N 4 , CrSi 2 As 4 , and CrGe 2 As 4 , which are ferromagnetic metals. In all, we found 21 semiconductors among the families of 32 and 34 valence electrons. 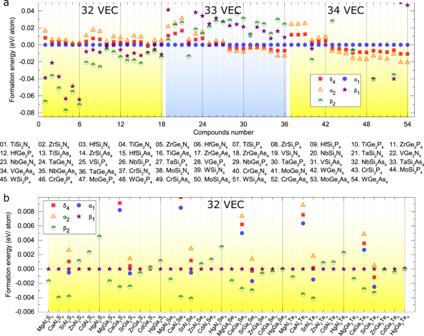Fig. 2: DFT-derived enthalpies of formation of MA2Z4monolayers. Here, we only show the data for the five lowest-energy configurations.aandbare forMbeing the first transition-metal group elements and alkali-earth elements, respectively. Ina,b, the enthalpies for each compound are relative to the total energies of theα1andβ1structures, respectively. Note that VEC is the number of valence electrons for one chemical formula. For more details about enthalpies of formation refer to Supplementary Tables2–7. We list the sizes of the bandgaps of all the semiconducting monolayers in Supplementary Table 2 , which are from both the standard DFT and HSE hybrid functional (HSE06) calculations. Besides, we have obtained many unexpected electronic properties for MA 2 Z 4 monolayers, such as nontrivial topological properties, 2D ferromagnetism, Ising superconductivity, and robust electron valleys with spin-momentum locking. In the following, we will discuss them in more detail. Systems with 32 valence electrons We first demonstrate that some of these systems exhibit nontrivial topological properties. We pay our attention to the family of MA 2 Z 4 (M = Mg, Ca, Sr, Zn, Cd, and Hg; A = Al and Ga; and Z = S, Se, and Te). Most of them are semiconductors. The semiconducting nature can be understood based on the structural properties and the chemical bonding in this type of system. In the InSe-like structure of the A 2 Z 2 monolayer, there is a covalent bond between the two A atoms. However, this bond is broken upon intercalating an MZ 2 monolayer into the A 2 Z 2 unit to form the intercalated system MA 2 Z 4 . Consequently, each atom tends to be charge compensated, which makes this system semiconducting. 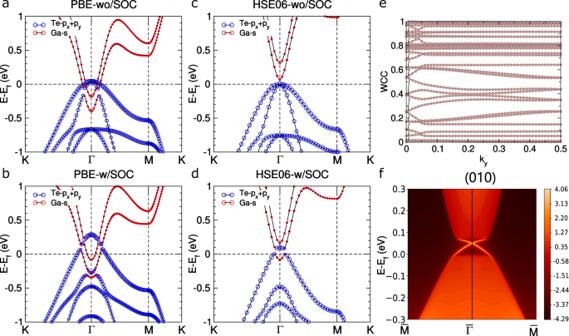Fig. 3: Topological properties ofβ2-SrGa2Te4. a,bThe band structures from standard DFT calculations without and with SOC, respectively.c,dThe results of HSE06 calculations without and with SOC, respectively. The bands are weighted by the orbital projections of Te and Ga.eThe evolution of the Wannier charge centers (WCC) in thekz= 0 plane.fEdge states ofβ2-SrGa2Te4for the HSE06 calculations. We have predicted a series of topological insulators in this family on the Perdew–Burke–Ernzerhof (PBE) level (Supplementary Table 3 ). For instance, our calculations show that β 2 -SrGa 2 Se 4 is a zero-gap semiconductor (Supplementary Fig. 8 ). Inclusion of spin–orbit coupling (SOC) leads to a gap opening of ~68 meV and band inversion at Γ. Our calculations see gapless states in this system and found that it has a value of Z 2 = 1. These results suggest that β 2 -SrGa 2 Se 4 is a topological insulator. We further investigate its topological properties by using the advanced HSE hybrid functional method. As a result, it becomes topologically trivial. In contrast, we found that β 2 -SrGa 2 Te 4 is topologically nontrivial by both the PBE and HSE06 methods. In Fig. 3 a, we show the electronic bands from PBE calculations without SOC, which indicates that this system has a metallic band structure. The inclusion of SOC induces a gap opening near Γ, which results in a separation of the valence and conduction bands (see Fig. 3 b). Similar to the case of β 2 -SrGa 2 Se 4 , we have Z 2 = 1 and gapless edge states. 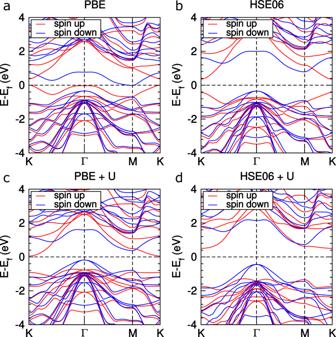Fig. 4: Band structures of ferromagneticδ4-VSi2P4under different methods. a,bPlots for PBE calculations with and without HubbardU.c,dCorresponding plots for HSE06 calculations. We then investigate the topological property by performing HSE06 calculations without and with SOC, of which the results are shown in Fig. 3 c, d, respectively. The calculation without SOC finds that there is a small direct bandgap at Γ. The inclusion of SOC induces a downward bending of the valence band at Γ, which signals the band inversion seen in the topological insulator Bi 2 Se 3 [38] . We further confirm this band inversion by the orbital-projected band structure shown in Fig. 3 d. We have also calculated the evolution of the Wannier charge centers, which also gives Z 2 = 1 (see Fig. 3 e). Moreover, we have observed gapless edge states for β 2 -SrGa 2 Te 4 (see Fig. 3 f) based on the Wannier functions obtained from the HSE06 calculations, which again confirms that this system is topologically nontrivial. Fig. 3: Topological properties of β 2 -SrGa 2 Te 4 . a , b The band structures from standard DFT calculations without and with SOC, respectively. c , d The results of HSE06 calculations without and with SOC, respectively. The bands are weighted by the orbital projections of Te and Ga. e The evolution of the Wannier charge centers (WCC) in the k z = 0 plane. f Edge states of β 2 -SrGa 2 Te 4 for the HSE06 calculations. Full size image Systems with 33 valence electrons These systems are in either the ferromagnetic state or the nonmagnetic state in this family. Among them, there are nine ferromagnetic systems, for which the magnetic configurations and the energetics are shown in Supplementary Fig. 9 and Supplementary Table 9 , respectively. Our standard PBE calculations found that among them, NbSi 2 N 4 and MGe 2 N 4 (M = V, Nb, and Ta) monolayers show a half-metallic behavior (Supplementary Fig. 5 ), whereas VSi 2 Z 4 (Z = N, P, and As) and VGe 2 Z 4 (Z = P and As) exhibit a gapless semiconducting behavior [50] , [51] . A close inspection of the PBE-derived band structure finds that the Fermi level of VSi 2 P 4 touches both the valence band maximum (VBM) and conduction band minimum (CBM), which are the spin majority and minority states, respectively (Fig. 4 a). In addition, we have calculated the magnetocrystalline anisotropy energy of VSi 2 P 4 , for which it is 56 μeV. This result indicates that its easy axis is out of plane. 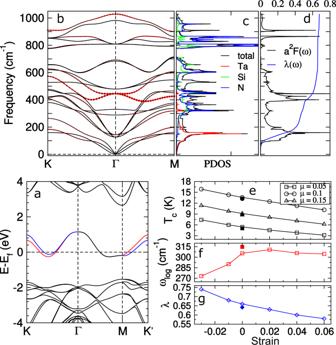Fig. 5: Ising superconductivity inα1-TaSi2N4. aContrasting spin splitting atKand\({K}^{\prime}\)forα1-TaSi2N4due to the SOC-induced Zeeman-like field. The red and blue lines represent different spin states.bPhonon dispersions andcphonon density of states ofα1-TaSi2N4.dEliashberg functionα2F(ω) and the electron–phonon coupling strengthλ(ω). Strain dependence ofethe superconducting transition temperature (Tc),flogarithmic average phonon frequency (ωlog), andgelectron–phonon coupling constant (λ). The solid symbols at the 0% strain denote the SOC-containing results. 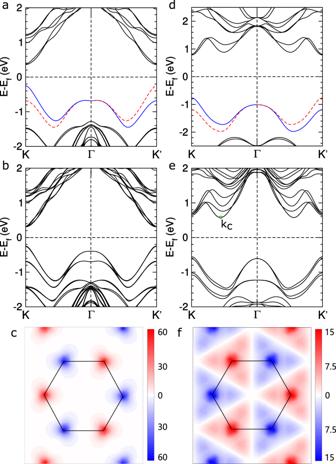Fig. 6: Comparison of electron valleys in betweenα2-WSi2P4and 2H-WSe2. a,dBand structure forα2-WSi2P4and 2H-WSe2monolayers. The blue and red lines represent different spin states.b,eBand structure for the bilayer ofα2-WSi2P4and 2H-WSe2.kcineindicates the CBM.d,fBerry curvature ofα2-WSi2P4and 2H-WSe2monolayers near theKand\({K}^{\prime}\)valleys. The black hexagons show the first Brillouin zones of the monolayers. Furthermore, our HSE06 calculation reveals that it is nearly a direct bandgap semiconductor (Fig. 4 b). We realized that the electron correlations related to the partially filled 3 d orbitals of the transition-metal atoms may be important for the band structure of such a kind of system. We then estimate the effective Coulomb interaction ( U ) by using the linear-response method [52] , which gives U = 4 eV for the V-3 d orbitals in VSi 2 P 4 . In Fig. 4 c, we show the band structure of VSi 2 P 4 from our PBE calculation with U (PBE + U ). One can see that inclusion of the Hubbard U opens a gap of ~0.3 eV, which is then increased up to ~1.0 eV by the HSE06 calculation (Fig. 4 d). Our calculations show that the HSE06 results are consistent with the PBE + U results that both predict a semiconducting behavior for the VSi 2 P 4 monolayer. Moreover, we make a comparison of the band structures for the HSE06 calculations with and without Hubbard U and found that the sizes of the predicted bandgaps are comparable, although there are visible differences in details of the electronic bands near K . Based on these observations, we then performed HSE06 calculations for all the ferromagnetic systems. As a result, they all show a sizable gap ranging from 0.2 to ~1.0 eV (Supplementary Fig. 5 ). Fig. 4: Band structures of ferromagnetic δ 4 -VSi 2 P 4 under different methods. a , b Plots for PBE calculations with and without Hubbard U . c , d Corresponding plots for HSE06 calculations. Full size image We use the Heisenberg spin Hamiltonian to understand the magnetic interactions in the VSi 2 P 4 monolayer. We extract the exchange interaction parameters between spins by fitting the total energies from our DFT calculations of various spin configurations to the Hamiltonian with the first nearest neighbors only, that is, H = − J ∑ < i j > S i ⋅ S j . We found that J is ~8 meV for S = 1. In fact, J 2 is negligibly small (<0.1 meV) if we fit the Hamiltonian up to the second nearest neighbors. Based on the magnetic exchange parameters, we obtain a Curie temperature of ~90 K by performing Metropolis Monte Carlo simulations of the Heisenberg Hamiltonian (Supplementary Fig. 11 ). The nonmagnetic systems of this family are metallic since they have one unpaired electron, which results in a half-filled electronic band (Supplementary Fig. 5 ). We note that among the systems, α 1 -TaSi 2 N 4 has a special band structure, that is, it has a disentangled band contributed by the Ta-5 d orbitals. Such a feature leads to the speculation of strong electron correlation in this system. Like in the case of VSi 2 P 4 , we have also carried out a linear-response calculation, which gives a value of ~2.5 eV for the U parameter of the Ta-5 d orbitals. Then, we investigate the effects of Hubbard U on the band structure of TaSi 2 N 4 and found that the half-filled band remains almost unchanged (Supplementary Fig. 12 ). Note that, in this system, the strong SOC along with the inversion symmetry breaking induces a large valley-contrasting spin splitting at K and K ′. Such a band structure favors the type-I Ising superconductivity, as already observed in NbSe 2 [12] . Following this inspiration, we have calculated the phonon spectrum and Eliashberg function ( α 2 F ( ω )) as well as derived the EPC strength ( λ ) for α 1 -TaSi 2 N 4 (Fig. 5 ). Using λ = 0.66 and the calculated logarithmic average phonon frequency of 305.58 cm −1 , we have derived a superconducting transition temperature of T c = 5.42–13.61 K via the Dynes modified McMillan formula with the effectively screened Coulomb repulsion constant of μ from 0.15 to 0.05. For α 2 -TaGe 2 P 4 , T c is ~3.75 K for μ = 0.1 (Supplementary Fig. 13 ). Moreover, we have examined the effects of SOC and strain on λ and T c of α 1 -TaSi 2 N 4 . We found that SOC has a minor effect on both λ and T c (see Fig. 5 g, e and Supplementary Fig. 13 ). We summarize our results of the strain effect (−3 to 6%) in Fig. 5 e, which show that T c varies nonlinearly with strain. T c is only reduced by ~32% under a large strain up to 6%. While T c is increased by ~24% under a compressive strain −3%. This trend indicates that the superconductivity in α 1 -TaSi 2 N 4 is robust against strain, which favors the observation of Ising superconductivity in the epitaxially grown monolayer. Fig. 5: Ising superconductivity in α 1 -TaSi 2 N 4 . a Contrasting spin splitting at K and \({K}^{\prime}\) for α 1 -TaSi 2 N 4 due to the SOC-induced Zeeman-like field. The red and blue lines represent different spin states. b Phonon dispersions and c phonon density of states of α 1 -TaSi 2 N 4 . d Eliashberg function α 2 F ( ω ) and the electron–phonon coupling strength λ ( ω ). Strain dependence of e the superconducting transition temperature ( T c ), f logarithmic average phonon frequency ( ω log ), and g electron–phonon coupling constant ( λ ). The solid symbols at the 0% strain denote the SOC-containing results. Full size image Systems with 34 valence electrons Among this family, we focus on Mo- and W-based MA 2 Z 4 (A = Si and Ge and Z = N, P, and As) monolayers. The reason is that some of them even show better electronic properties than the dichalcogenide counterparts of Mo and W, that is, the TMDs monolayers. For the nitrides, that is, MSi 2 N 4 and MGe 2 N 4 (M = Mo and W), the lowest-energy structures are in the α 1 phase, whereas for the phosphides and arsenides, the α 2 structure becomes favorable. Despite this difference, the inversion symmetry is absent in both structures. Among these systems, MoSi 2 P 4 , MoSi 2 As 4 , WSi 2 P 4 , and WSi 2 As 4 are predicted to be direct bandgap semiconductors by both the PBE and HSE06 calculations. One prominent feature of the band structure is that like the TMDs monolayers, there are electron valleys at K and \({K}^{\prime}\) [53] . The strong atomic SOC in Mo and W induces large spin splittings at K and \({K}^{\prime}\) . For α 2 -WSi 2 P 4 (Fig. 6 a), the spin splitting at K is ~0.4 eV, which is comparable to that of 2 H -WSe 2 monolayer [54] , [55] . In addition, the strong SOC together with the inversion symmetry breaking gives rise to spin-momentum locking at the valleys and a Berry curvature contrasting at the two valleys (see Fig. 6c ). These features provide opportunities for exploring the spin-valley physics and manipulating their electronic properties via doping, interfacing, and layer stacking including Morie patterns [56] , [57] . Fig. 6: Comparison of electron valleys in between α 2 -WSi 2 P 4 and 2 H -WSe 2 . a , d Band structure for α 2 -WSi 2 P 4 and 2 H -WSe 2 monolayers. The blue and red lines represent different spin states. b , e Band structure for the bilayer of α 2 -WSi 2 P 4 and 2 H -WSe 2 . k c in e indicates the CBM. d , f Berry curvature of α 2 -WSi 2 P 4 and 2 H -WSe 2 monolayers near the K and \({K}^{\prime}\) valleys. The black hexagons show the first Brillouin zones of the monolayers. Full size image The unique structural and electronic structures of our systems show advantages over the TMDs layers in several aspects. First, the electron valleys in them are robust against interlayer interactions. In the case of the TMDs bilayers, by the layer hybridization, the conduction band at Γ is pushed up to a higher energy and the valence band at k c is pushed down to a lower energy than that at K and \({K}^{\prime}\) (see Fig. 6 e and Supplementary Fig. 15 ), resulting in a direct–indirect bandgap transition. Note that there is a large energy difference between the VBM at K ( \({K}^{\prime}\) ) and Γ for α 2 -WSi 2 P 4 . Moreover, the valence band and conduction band are dominated by the d -orbitals of W (Mo) (Supplementary Fig. 16 ), which is sandwiched by double-atomic AZ layers. Therefore, the VBM and CBM can be less affected by interfacing and layer stacking than those of the TMDs layers. In Fig. 6 b, we show the band structure of the α 2 -WSi 2 P 4 bilayer. One can see that the nature of the direct bandgap is maintained well upon the layer stacking. In addition, we found that α 2 -WSi 2 P 4 exhibits a large hole mobility of up to 460 cm 2 V −1 s −1 and an electron mobility of about 150 cm 2 V −1 s −1 (see Supplementary Fig. 17 and Supplementary Table 8 ). These values are ~150% of those for the 2 H -WSe 2 monolayer [58] , [59] , indicating that α 2 -WSi 2 P 4 may have better electronic transport properties than the TMDs monolayers. In summary, we have presented an intercalation approach to construct septuple-atomic-layer MA 2 Z 4 monolayers. We have illustrated this strategy by performing first-principles calculations for systems with 32–34 valence electrons. Our calculations predict that among 90 candidates, 72 compounds are both thermodynamically and dynamically stable. The systems with 32 and 34 valence electrons are mostly semiconductors, whereas those with 33 valence electrons are either nonmagnetic metals or ferromagnetic semiconductors. In addition, we found that these systems exhibit a number of novel electronic properties. In particular, β 2 -SrGa 2 Te 4 is found to be a topological insulator by both the PBE and HSE06 calculations. In addition, our study finds that among the family of the systems with 33 valence electrons, the V-based MA 2 Z 4 monolayers are basically ferromagnetic semiconductors as revealed by our HSE06 calculations. As for the nonmagnetic metals like α 1 -TaSi 2 N 4 in this family, the inversion symmetry breaking and the strong SOC lead to a valley-contrast spin splitting in the half-filled band with out-of-plane spin polarizations. We further predict that such features favor the type-I Ising superconductivity in α 1 -TaSi 2 N 4 . Moreover, our study reveals that α 1 -WSi 2 P 4 not only has a direct bandgap with robust electron valleys against layer interactions but also shows superior electronic transport properties compared to the TMDs monolayer WSe 2 . Finally, we would like to emphasize that our currently proposed intercalated architecture approach can be indeed extended to MA 2 Z 4 monolayer materials with M for late transition metal elements, such as MnBi 2 Te 4 for which our current calculations also correctly capture the agreements to experiments. Furthermore, it can be generalized to a wider way. For instance, n =7 MA 2 Z 4 monolayer materials can be constructed by intercalating n = 2 silicene-like monolayer into n = 5 Bi 2 Se 3 -like monolayer and, we can also even combine n = 3 MoS 2 -like monolayer and n = 5 Bi 2 Se 3 -like monolaye to form new type n = 8 monolayer materials, and so on. Our study thus provides an effective way of designing septuple layer systems with unusual electronic properties. Electronic and phononic band structures First-principles calculations were performed by applying the Vienna ab initio simulation package (VASP) [60] , [61] , and the PBE exchange-correlation functional was used to calculate the enthalpy of formation and band structure. To further get a more accurate bandgap, a hybrid function (HSE06) was applied. The plane-wave energy cutoff was adopted to be ranging from 250 eV (MgGa 2 Te 4 ) to 500 eV (MoSi 2 N 4 ). The 2D Brillouin zone was sampled by a 15 × 15 k -mesh for the self-consistent calculations. Structural relaxations were done with a threshold of 10 −3 eV Å −1 for the residual force on each atom. The energy convergence criteria were set as 10 −6 eV. To minimize the interactions between the monolayer and its periodic images, a vacuum of 20 Å was used for all the calculations. Phonon dispersions were obtained using density functional perturbation theory and Phonopy package [62] . We used a large supercell (either a 4 × 4 supercell or a 5 × 5 supercell) for the force calculations. EPC and superconductivity For metallic materials, the EPC constant λ is given by [63] 
    λ =2∫dωα^2F(ω )/ω
 (1) where α 2 F ( ω ) is the Eliashberg function, which is defined as 
    α^2F(ω )=1/2π N(ϵ_F)∑ _qνδ (ω -ω_qν)γ_qν/ℏω_qν,
 (2) where N ( ϵ F ) is the density of states at the Fermi level, ω q ν is the phonon frequency of the mode ν at wavevector q and γ q ν is the phonon linewidth or lifetime. The Eliashberg function α 2 F ( ω ) is used to calculate logarithmic average phonon frequencies by \(\omega_{\mathrm{log}} = {\mathrm{exp}} \left[\frac{2}{\lambda }\int_{0}^{\infty }\frac{{\mathrm{d}}\omega }{\omega }{\alpha }^{2}F (\omega ){\mathrm{log}}\,\omega \right]\) . We use the Allen–Dynes-modified McMillan formula to estimate the superconducting transition temperature [64] , that is, \({T}_{\mathrm{c}}=\frac{\omega_{\mathrm{log}}}{1.2}{\mathrm{exp}} \left[\frac{-1.04 ( 1+ \lambda )}{\lambda -{\mu }^{* } (1 + 0.62\lambda )}\right]\) . The above calculations were performed using the Quantum-ESPRESSO package with ultrasoft pseudopotentials and local-density approximation exchange-correlation functional [52] , [65] . For α 1 -TaSi 2 N 4 , the kinetic energy cutoff and charge density cutoff of the plane-wave basis are 60 and 480 Ry, respectively. A 32 × 32 k -mesh with Marzari–Vanderbilt cold smearing of 0.02 Ry is used for self-consistent calculations. A 4 × 4 q -mesh is used to obtain dynamic matrix and EPC constant, respectively. For α 2 -TaGe 2 P 4 , a kinetic energy cutoff of 80 Ry and a charge density cutoff of 640 Ry are used. A 36 × 36 k -mesh and 6 × 6 q -mesh are used to calculate EPC constant and the superconducting T c . Carrier mobility The intrinsic carrier mobility μ of 2D materials was derived based on the deformation potential (DP) approximation [66] 
    μ_2D=2eℏ^3C/3k_BT|m^* |^2E_1^2,
 (3) where C is the elastic modulus defined as \(\left[{\partial }^{2}E/\partial {\delta }^{2}\right]/{S}_{0}\) , m * is the effective mass at the CBM or VBM, and T is the temperature. Here, room temperature T = 300 K was used. E 1 is the DP constant defined as \({{\Delta }}E/\left({{\Delta }}l/{l}_{0}\right)\) , where Δ E is the change of the eigenvalue at CBM or VBM and Δ l is the lattice dilation along deformation direction. Calculation of the enthalpy of formation The enthalpy of formation of a MA 2 Z 4 monolayer (per atom) can be expressed as: 
    E_f={E_tot-(E_M+2E_A+4E_Z)}/7,
 (4) where E tot is the total energy of the system, and E M , E A , and E Z are the ground state total energies of the elementary crystals of M, A, and Z, respectively. Calculations of Berry curvature and the Z 2 topological invariant The Berry curvature of a 2D material with n bands can be defined as [67] , [68] , [69] : 
    Ω_z(k)=∇_k× i⟨u_n,k| ∇_ku_n,k⟩ ,
 (5) where u n , k is the lattice periodic part of the Bloch wave functions. Our calculations were performed using the Wannier90 package [70] , which constructs u n , k via an ab initio tight-binding method on the basis of maximally localized Wannier functions. The values of the topological invariant Z 2 were obtained by calculating the Wannier charge centers [71] . The edge states were obtained using an iterative Green functions method [72] . The above calculations were based on the ab initio tight-binding parameters from the Wannier90 calculations.